O2evolution and recovery of the water-oxidizing enzyme In photosystem II, light-induced water oxidation occurs at the Mn 4 CaO 5 cluster. Here we demonstrate proton releases, dioxygen formation, and substrate water incorporation in response to Mn 4 CaO 5 oxidation in the protein environment, using a quantum mechanical/molecular mechanical approach and molecular dynamics simulations. In S 2 , H 2 O at the W1 site forms a low-barrier H-bond with D1-Asp61. In the S 2 -to-S 3 transition, oxidation of O W1 H – to O W1 •– , concerted proton transfer from O W1 H – to D1-Asp61, and binding of a water molecule W n -W1 at O W1 •– are observed. In S 4 , W n -W1 facilitates oxo-oxyl radical coupling between O W1 •– and corner μ-oxo O4. Deprotonation via D1-Asp61 leads to formation of O W1 =O4. As O W1 =O4 moves away from Mn, H 2 O at W539 is incorporated into the vacant O4 site of the O 2 -evolved Mn 4 CaO 4 cluster, forming a μ-oxo bridge (Mn3–O W539 –Mn4) in an exergonic process. Simultaneously, W n -W1 is incorporated as W1, recovering the Mn 4 CaO 5 cluster. Dioxygen can be produced by removing four electrons and four protons from two substrate water molecules: 2H 2 O → O 2 + 4 H + + 4e – . In a protein-pigment complex photosystem II (PSII), the water-oxidation reaction proceeds at the oxygen-evolving complex via the S n -state transitions ( n represents the total number of oxidation steps) [1] , [2] , [3] . The oxygen-evolving complex is linked with electron transfer pathways, proton transfer pathways, and substrate water intake pathways. Excitation of P680, which is composed of four chlorophyll a molecules, leads to electron transfer to the second plastoquinone, Q B , via pheophytin a and the first plastoquinone, Q A . The resulting P680 •+ state is stabilized by electron transfer from the Mn 4 CaO 5 cluster via redox active D1-Tyr161 (TyrZ) (Fig. 1 ). Fig. 1 Proton and electron transfer pathways near Mn 4 CaO 5 . Blue and pink arrows indicate proton and electron transfer pathways proceeding from the Mn 4 CaO 5 cluster, respectively Full size image Protons released from substrate water molecules are transferred via proton transfer pathways (e.g., O4-water chain [4] ), which proceeds from the Mn 4 CaO 5 cluster toward the protein bulk surface (Fig. 1 ). The releases of protons are observed with a typical stoichiometry of 1:0:1:2 for the S 0 → S 1 → S 2 → S 3 → S 0 transitions, respectively [5] . The O4-water chain is a chain of water molecules, which forms an H-bond with the O4 site of the Mn 4 CaO 5 cluster via a water molecule W539 [4] . Since the rate constant is pH-independent in the S 0 -to-S 1 transition, the absence of ionizable groups in the O4-water chain fits with the suggestion that the O4-water chain is the relevant proton transfer pathway [5] , [6] . Although release of a proton is not observed in the S 1 -to-S 2 transition, it seems likely that migration of a proton or internal proton transfer can occur (e.g., ref. [7] ). On the other hand, the rate constant for the S 2 -to-S 3 transition is pH-dependent, which suggests that ionizable groups are involved in the proton-transfer pathway [5] , [8] . Ionizable groups that are not ligands near the Mn 4 CaO 5 cluster are D1-Asp61 and CP43-Arg357 [9] . In the S 3 -to-S 0 transition, O–O bond formation and release of O=O occur. The rate constant of 1–2 ms involved in the S 3 -to-S 0 transition is pH-independent with a kinetic isotope effect ( k D / k H ) of 1.4 [6] , and may correspond to O 2 release and incorporation of a substrate water molecule [6] , [10] . k D / k H = 1.4 is also typical for alteration in the H-bond pattern along water chains before and after proton transfer (pre-PT and post-PT H-bond patterns, respectively) in the Grotthuss mechanism [11] . Once proton transfer occurs, the pre-PT pattern transforms to the post-PT pattern [4] . The slow-exchanging and fast-exchanging water molecules are candidate substrates in the Mn 4 CaO 5 cluster [12] . In the S 0 -to-S 1 transition, the exchange rate of the slow-exchanging water molecule decreases 600 times [12] and deprotonation of the slow-exchanging water molecule may occur, indicating that it may be a μ-OH bridge of the Mn 4 CaO 5 cluster in S 0 [13] . In the S 1 -to-S 2 transition, the exchange rate of the slow-exchanging water molecule increases 100 times [12] . The exchange rate of the fast-exchanging water molecule decreases three times in the S 2 -to-S 3 transition [14] . The fast-exchanging water molecule may be a terminal ligand to Mn[2] and possibly form an H-bond with D1-Asp61 [13] , [15] . The corresponding water molecule is W1 in the crystal structure analyzed at 1.9 Å resolution [9] . These water molecules approach the catalytic site from the bulk region via water channels. The D1-Glu65/D2-Glu312 channel is a candidate substrate water intake channel. The D1-Glu65/D2-Glu312 channel provides water molecules near TyrZ and the Mn 4 CaO 5 cluster. It can also deliver water molecules to the W539 and W538 sites in the O4-water chain via D1-Asp61 [16] . Recently, the two-flash illuminated PSII structure analyzed at 2.35 Å resolution was reported, demonstrating several characteristic O sites in the Mn 4 CaO 6 moiety [17] (e.g., W538, W539, O4, and O6). W538 [9] (i.e., W665 [17] ) was unambiguously identified in both the 1.9 Å [9] and radiation-damage-free [18] PSII crystal structures [4] , whereas it was absent in the two-flash illuminated PSII structure. W538 forms an H-bond with W539. The averaged O4…O W539 (i.e., O4…O W567 [17] ) distance of 2.32 Å identified in the two-flash illuminated PSII structure is exceptionally short in comparison with the typical O–O distances of ~2.8 Å for standard (asymmetric) H-bonds in H 2 O. The two-flash illuminated PSII structure shows the presence of O6 near O5. The O6…O5 distance is 1.5 Å, which is close to the distance for peroxide (O–O) 2– . This suggests that formation of O=O may occur at this site, which fits the reaction model proposed by Siegbahn et al. [19] . On the other hand, it is unclear whether the reaction model could also explain how the other characteristic O sites (e.g., W538, W539, and O4) are involved in the mechanism of water oxidation. It should be noted that the B -factor values of these O atoms are at the same level in the two-flash illuminated PSII structure. Here we analyzed alterations in the Mn 4 CaO 5 structure and H-bond/water network in response to Mn 4 CaO 5 oxidation in the PSII protein environment, using a quantum mechanical/molecular mechanical (QM/MM) approach and molecular dynamics (MD) simulations based on the PSII crystal structure. In S 2 , the proton of H 2 O at W1 significantly migrates toward D1-Asp61 due to oxidation of Mn4, forming a low-barrier H-bond (HO W1 – …H + … – OOC D1-Asp61 ). In the S 2 -to-S 3 transition, oxidation of O W1 H – to O W1 •– preferentially occurs with respect to oxidation of Mn1(III) to Mn1(IV), because D1-Asp61 accepts the proton from O W1 H – and facilitates oxidation to O W1 •– via proton-coupled electron transfer (i.e., decreasing the redox potential of W1 for oxidation). In S 3 , a water molecule binds at O W1 •– . Incorporation of water molecules (including W2 and W3) into the open-cubane O5 site are not observed. Since the nearest μ-oxo to O W1 •– is O4, oxo-oxyl radical coupling occurs between O4 and O W1 •– in S 4 , resulting in (O W1 –O4) 2– formation. As O W1 =O4 moves away from the Mn3/Mn4 moiety, H 2 O at W539 is incorporated into the vacant O4 site near CP43-Arg357, forming a μ-oxo bridge with Mn3–O W539 and Mn4–O W539 in a concerted exergonic process. Incorporation of W539 into the O4 site requires reorientation of W539, which induces alterations in the H-bond pattern from the post-PT pattern to pre-PT pattern along the O4-water chain. A water molecule, which binds at O W1 •– in S 3 , is also incorporated into the vacant W1 site (i.e., new W1), recovering the Mn 4 CaO 5 cluster. Formation of a low-barrier H-bond between W1 and D1-Asp61 We used the deprotonated open-cubane S 2 structure, where (Mn1,Mn2,Mn3,Mn4) = Mn(III,IV,IV,IV), as it seems to be energetically more stable than the closed-cubane S 2 structure [20] , [21] , [22] , [23] . The p K a of H-bond donor and acceptor moieties in H-bonds can be analyzed from the potential-energy profiles of the H-bonds [24] , [25] , [26] . In H-bonds, a proton is more likely to populate the moiety with the higher p K a value between the two moieties [26] . The energy difference between the H-bond donor and acceptor moieties corresponds to the p K a difference and this feature also holds true for H-bonds in protein environments [27] . QM/MM calculations showed that a short H-bond between H 2 O at W1 and D1-Asp61 (O W1 …O D1-Asp61 = 2.45 Å) was formed in the open-cubane S 2 (Fig. 2a ). The potential-energy profile suggested that the O W1 …O D1-Asp61 H-bond is a low-barrier H-bond (LBHB, where the p K a difference for the donor and acceptor moieties is nearly zero [25] , [27] ) (Fig. 2b ), and that the proton is significantly migrated toward D1-Asp61 and delocalized over the two moieties already in S 2 (Fig. 2a ). This may correspond to the significant changes in the H-bond properties between D1-Asp61 and a water molecule in the S 1 -to-S 2 transition observed in Fourier transform infrared (FTIR) spectroscopy [7] . 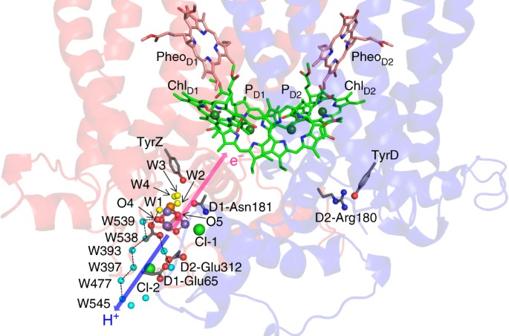Fig. 1 Proton and electron transfer pathways near Mn4CaO5. Blue and pink arrows indicate proton and electron transfer pathways proceeding from the Mn4CaO5cluster, respectively It should also be noted that the spin configurations (e.g., high, low, ferromagnetic, and antiferromagnetic) did not essentially affect the resulting optimized Mn 4 CaO 5 geometry and energies in the present case (Table 1 ). Potential-energy profiles also remained unaffected since proton transfer does not involve oxidation of Mn ions (Supplementary Figure 1 ). Fig. 2 The open-cubane S 2 -to-S 3 transition. a QM/MM geometries. Mn, Ca, O, and H atoms are represented by purple, orange, red, and black balls, respectively. Dotted lines indicate distances (excluding H atoms). b The energy profiles of the H-bonds between W1 (H 2 O/OH – ) and D1-Asp61 in S 2 and W1(OH • /O •– ) and D1-Asp61 in S 3 . The black curve corresponds to release of the proton from H 2 O at W1 to D1-Asp61 in S 2 , whereas the red curve corresponds to release of the proton from OH • at W1 to D1-Asp61 in S 3 . The spin configurations (e.g., high, low, ferromagnetic, and antiferromagnetic) did not essentially affect the resulting optimized Mn 4 CaO 5 geometries and potential-energy profiles (Table 1 and Supplementary Figure 1 ) Full size image Table 1 Spin configurations and the resulting optimized Mn 4 CaO 5 geometries (in Å) and energies (in kcal/mol) calculated for antiferromagnetically coupled Mn ions with respect to ferromagnetically coupled Mn ions in S 2 Full size table Absence of Mn oxidation in the S 2 -to-S 3 transition Unexpectedly, oxidation of S 2 to S 3 did not involve oxidation of Mn; however, oxidation of O W1 H – to O W1 •– and concerted proton transfer from O W1 H – to D1-Asp61 did occur, resulting in Mn(III,IV,IV,IV)…O W1 •– …HOOC D1-Asp61 in the open-cubane conformation (Fig. 2a ). Accordingly, the first proton of W1 (from H 2 O/OH – ), which was delocalized over the low-barrier O W1 …H + …O D1-Asp61 bond in S 2 , seems likely to have been released toward the bulk surface via D1-Asp61 (along the D1-Glu65/D2-Glu312 water channel) in the S 2 -to-S 3 transition [16] , [28] , since the potential-energy profile indicated that even the second proton from W1 (from OH • /O •– ) can be released to D1-Asp61 (Fig. 2 ). 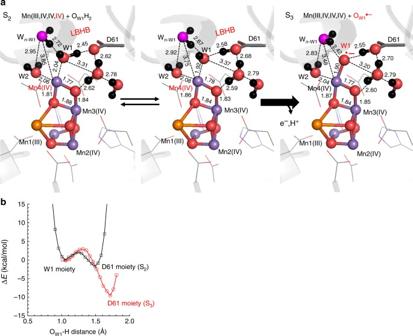Fig. 2 The open-cubane S2-to-S3transition.aQM/MM geometries. Mn, Ca, O, and H atoms are represented by purple, orange, red, and black balls, respectively. Dotted lines indicate distances (excluding H atoms).bThe energy profiles of the H-bonds between W1 (H2O/OH–) and D1-Asp61 in S2and W1(OH•/O•–) and D1-Asp61 in S3. The black curve corresponds to release of the proton from H2O at W1 to D1-Asp61 in S2, whereas the red curve corresponds to release of the proton from OH•at W1 to D1-Asp61 in S3. The spin configurations (e.g., high, low, ferromagnetic, and antiferromagnetic) did not essentially affect the resulting optimized Mn4CaO5geometries and potential-energy profiles (Table1and Supplementary Figure1) MD simulations indicated that D1-Asp61 was able to accept a proton by rotating the protonated O site (Supplementary Figure 2 ), as reported in QM/MM-MD simulations by Narzi et al. [29] . Since p K a (OH – / O 2– ) ( = 24) > p K a (OH • / O •– ) (=12 [30] ), the concerted oxidation and proton release of O W1 H – to O W1 •– occurs without stabilizing O W1 H • on Mn4(IV). In the S 2 -to-S 3 transition, it remains unclear whether a Mn-centered oxidation (e.g., ref. [31] ) or a ligand-centered oxidation (e.g., ref. [32] ) occurs (discussed in refs. [5] , [13] , [33] , [34] ). Some theoretical studies favor the Mn-centered oxidation model over the ligand-centered oxidation model (e.g., refs. [35] , [36] , [37] , [38] , [39] ). Recent electrochemical analysis using the α-MnO 2 electrode shows that addition of carboxylic acid (benzoic acid) induced proton-coupled electron transfer, resulting in a decrease in the redox potential required for water oxidation and an increase in evolved O 2 at lower potentials [40] . Remarkably, FTIR spectra suggest that benzoic acids do not directly ligate to the Mn ion but form an H-bond with a ligand water molecule of the Mn ion, as identified in the Mn4…W1…D1-Asp61 moiety in PSII. The presence of benzoic acid as the proton acceptor facilitates proton-coupled electron transfer and can avoid accumulation of the positive charge in response to oxidation of Mn, leading to a decrease in the redox potential required for oxidation of water [40] . This may hold true for the present case, where proton-coupled electron transfer from W1 to D1-Asp61 occurs in response to the S 2 -to-S 3 transition, which can specifically decrease the redox potential of W1 for one-electron oxidation. The absence of the Mn-centered oxidation in the S 2 -to-S 3 transition has been reported in spectroscopic studies by Messinger et al. ; Mn was not oxidized, but a ligand substrate molecule was oxidized in the S 2 -to-S 3 transition and an O radical was present in S 3 (Mn(III)Mn(IV) 3 ) [32] , which is consistent with the present results. It should be noted that although TyrZ and the H-bond network were also considered quantum-chemically (i.e., in the QM region), we did not observe formation of TyrZ • . According to the interpretation of FTIR difference spectroscopy, a water molecule was incorporated into the Mn 4 CaO 5 moiety in the S 2 to S 3 transition [41] . In S 3 , MD simulations showed that a water molecule existed near W1 (W n -W1 ) and could form an H-bond with O W1 •– (Fig. 3 ). The corresponding water molecule is absent in the PSII crystal structures [9] , [18] . The binding of W n -W1 seems to be made more pronounced by the negatively charged O W1 •– in S 3 (Supplementary Table 1 ). Near W n -W1 there exists D1-Ser169, which has been proposed to provide access to water molecules for the substrate-binding site [42] . QM/MM calculations also showed that the H-bond between W1 and W n -W1 is remarkably short: 2.42 Å in S 3 (i.e., O •– at W1; Fig. 2a ) compared with 2.72 Å in S 2 (i.e., H 2 O at W1; Fig. 2a ). MD simulations suggested that water molecules at the W n -W1 binding moiety are exchangeable with bulk water via the D1-Glu65/D2-Glu312 water channel [16] , indicating that the D1-Glu65/D2-Glu312 water channel can serve as the intake channel for W n -W1 . Fig. 3 Water distribution near the Mn 4 CaO 5 cluster. a Water distribution in S 3 after an equilibrating MD run at 45−50 ns (250 snapshots). The position of W n -W1 is indicated by the dotted circle. b The corresponding view in the QM/MM-optimized geometry in S 3 . Dotted black lines indicate interactions. c Water distribution in S 1 after an equilibrating MD run at 45−50 ns (250 snapshots). W n -W1 is absent in S 1 (dotted circle) Full size image We did not observe any incorporation of water molecules (including W2 and W3) into the open-cubane O5 site, nor did we observe formation of O W2 •– in QM/MM calculations, because of the absence of the proton acceptor groups (e.g., D1-Asp61). Below, we focus on the Mn 4 CaO 5 cluster based on the obtained open-cubane S 3 with O W1 •– . Oxidation of S 3 and formation of (O W1 –O4) 2– Oxidation of S 3 resulted in Mn(IV,IV,IV,IV)…O W1 •– …HOOC Asp61 (we denote the oxidized S 3 states as “S 4 ”, Fig. 4a ). The presence of O W1 •– in S 4 suggests that W1 may be involved in O–O single-bond formation via oxo-oxyl radical coupling. The nearest μ-oxo to O W1 •– is O4. Since we observed neither formation of O W2 •– nor a reactive Mn(V)=O species, we focused on O W1 •– and O4. Fig. 4 The S 4 and pre-S 0 states. a QM/MM geometries. Mn, Ca, O, and H atoms are represented by purple, orange, red, and black balls, respectively. Dotted lines indicate distances (excluding H atoms). Release of (O W1 –O4) •– from the Mn3/Mn4 moiety (i.e., the Mn3…O4 distance was increased) resulted in formation of O W1 =O4. See supplementary Figure 4 for the energy profile. 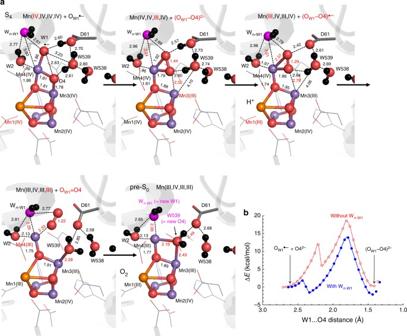Fig. 4 The S4and pre-S0states.aQM/MM geometries. Mn, Ca, O, and H atoms are represented by purple, orange, red, and black balls, respectively. Dotted lines indicate distances (excluding H atoms). Release of (OW1–O4)•–from the Mn3/Mn4 moiety (i.e., the Mn3…O4 distance was increased) resulted in formation of OW1=O4. See supplementary Figure4for the energy profile.bThe energy profiles of the (OW1–O4)2−formation (the first and second panels ina) in the presence (blue curve) and absence (red curve) of Wn-W1. The initial lower barriers correspond to reorientation of the carboxylate group of D1-Asp61 with respect to OW1•–/(OW1–O4)2– b The energy profiles of the (O W1 –O4) 2 − formation (the first and second panels in a ) in the presence (blue curve) and absence (red curve) of W n -W1 . The initial lower barriers correspond to reorientation of the carboxylate group of D1-Asp61 with respect to O W1 •– /(O W1 –O4) 2– Full size image The potential-energy profile suggests that as oxo-oxyl radical coupling (e.g., ref. [43] ) proceeds between O4 and O W1 •– , formation of (O W1 –O4) 2– (confirmed by O W1 –O4 = 1.44 Å and the spin density (2 S ) = 0 for both O W1 and O4) and concerted electron transfer from the (O W1 –O4) moiety to Mn3 occur, resulting in Mn(IV,IV,III,IV)…(O W1 –O4) 2– …HOOC Asp61 (Fig. 4a ). The energy barrier for the (O W1 –O4) 2– formation was 13.9 kcal/mol (Fig. 4b ), which is essentially consistent with the estimated values (e.g., 12.1 kcal/mol [44] ). 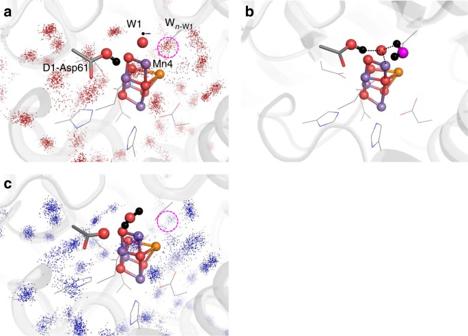In all S-state transitions, including the (O W1 –O4) 2– formation process, Mn2(IV) is not involved in oxidation/reduction, which could explain the similar energy barriers in the antiferromagnetically (↑↓↑↑) (Fig. Fig. 3 Water distribution near the Mn4CaO5cluster.aWater distribution in S3after an equilibrating MD run at 45−50 ns (250 snapshots). The position of Wn-W1is indicated by the dotted circle.bThe corresponding view in the QM/MM-optimized geometry in S3. Dotted black lines indicate interactions.cWater distribution in S1after an equilibrating MD run at 45−50 ns (250 snapshots). Wn-W1is absent in S1(dotted circle) 4 ) and ferromagnetically (↑↑↑↑) (Supplementary Figure 3 ) coupled forms. The energy barrier was 18.6 kcal/mol in the absence of W n -W1 (Fig. 4b and Supplementary Figure 3 ). Because W n -W1 lowers the energy barrier, it may serve as a catalyst for (O W1 –O4) 2– formation in S 4 . As formation of (O W1 –O4) 2– proceeded, the H atom of W n -W1 , which was initially oriented toward O W1 •– , became oriented away from (O W1 –O4) 2– . Simultaneously, the W n -W1 …Mn4 distance decreased from 3.60 to 3.24 Å, owing to displacement of W1 toward O4, allowing W n -W1 to approach Mn4 (Fig. 4 ). Formation of O W1 =O4 When D1-Asp61 was deprotonated in the presence of (O W1 –O4) 2– , QM/MM calculations resulted in formation of (O W1 –O4) •– (e.g., ref. [45] , confirmed by O W1 –O4 = 1.29 Å and the spin density (2 S ) = 0.8 for O W1 and 0.4 for O4) and concerted electron transfer to Mn1 (Fig. 4 ). Furthermore, the following events occurred concertedly: (i) W n -W1 approached Mn4, (ii) (O W1 –O4) •– moved away from Mn3/Mn4, (iii) W539 approached Mn3, and (iv) electron transfer from (O W1 –O4) •– to Mn4 occurred, resulting in formation of O W1 =O4 (confirmed by O W1 –O4 = 1.22 Å and the spin density (2 S ) = 1.0 for O W1 and 0.9 for O4; Fig. 4 ) in an exergonic process (Supplementary Figure 4 ). The resulting oxidation state was Mn(III,IV,III,III), returning to an Mn oxidation state identical to that of S 0 [4]. After O 2 evolution, the O 2 -evolved Mn 4 Ca“O 4 ” cluster formed, which resembled the O4-lacking Mn 4 CaO 4 cluster reported in the 3.5-Å PSII crystal structure [46] and the O4-lacking synthetic Mn 4 CaO 4 cluster reported by Zhang et al. [47] . The evolved O 2 molecule is present in the hydrophobic space between Mn4 and D1-Ile60 (next to D1-Asp61), which has been proposed to serve as an O 2 -exiting pathway [48] . Indeed, O 2 evolution was significantly lowered when D1-Ile60 was mutated to bulky phenylalanine [49] . Release of O 2 and incorporation of W539 into the O4 site Intriguingly, when evolved O 2 was absent near Mn3/Mn4, QM/MM calculations resulted in exergonic incorporation of H 2 O at W539 (in the O4-water chain [4] , Fig. 1 ) into the vacant O4 site of the Mn 4 CaO 4 cluster and formation of a μ-oxo bridge with Mn3–O W539 (2.43 Å) and Mn4–O W539 (2.19 Å) (pre-S 0 state, Fig. 4 ). While W539 was incorporated into the Mn 4 CaO 4 cluster, W n -W1 simultaneously approached Mn4 and was incorporated into the Mn 4 CaO 5 cluster as the new W1 ligand (W n -W1 …Mn4 = 2.08 Å). The resulting QM/MM geometry (Fig. 4 ) was quite similar to that of the original PSII crystal structure, demonstrating the ability to recover the initial state in the Kok cycle. D1-Asp61, the only acidic residue that is not a ligand near the Mn 4 CaO 5 cluster (i.e., a second sphere ligand), accepted an H-bond from W539, delocalizing the negative charge over [D1-Asp61…W539] – and inducing O W539 δ– . Thus, D1-Asp61 provides a driving force for the incorporation (i.e., it facilitates interactions between O W539 δ– and Mn3(III)/Mn4(III)) (Fig. 5 ). Indeed, it has been reported that O 2 release was dramatically decelerated in the D1-D61N mutant [50] , [51] , [52] . As long as O 2 was present in the Mn3/Mn4 moiety, H 2 O at W539 did not incorporate into the O4-binding site (Supplementary Figure 4 ), i.e., the presence of O 2 at the Mn3/Mn4 moiety sterically inhibited incorporation of H 2 O at W539 into the O4 site. Therefore, the exergonic incorporation of W539, which was facilitated by D1-Asp61, could contribute to expulsion of O 2 (Supplementary Figure 4 ). Fig. 5 Difference in the orientations and interactions of the incorporating H 2 O molecule. a The O4 site. Anionic D1-Asp61 attracts the H δ+ and orients the O δ– of the incorporating H 2 O toward cationic Mn3(III), Mn4(III), and CP43-Arg357, resulting in attraction. b The O5 site. The absence of an anionic H-bond acceptor and the nature of the incorporating H 2 O as a ligand of Mn4 force the H δ+ of the incorporating H 2 O to face cationic Mn1(III), Mn3(III), and Mn4(III), resulting in repulsion. The absence of D1-Asp61 near O5 would be energetically disadvantageous for incorporating H 2 O into the O5 site. O4 is located at the “corner” of the Mn3–O4 and O4–Mn4 bonds. Due to the presence of D1-Asp61, O W539 δ– can always be oriented toward the vacant O4 site, which makes incorporation energetically favorable (Supplementary Figure 4a ). On the other hand, if W2 is incorporated into the center of the Mn1–(O5)–Mn4 bond, H W2 δ+ is oriented toward cationic Mn1(III) and Mn4(III), causing repulsion (Supplementary Figure 4b ). Indeed, QM/MM calculations show that neither W2 nor W3 was incorporated into the vacant O5 site of the O5-depleted Mn 4 CaO 4 cluster. Depletion of O5 did not even affect the H-bond network near O5, including the short low-barrier H-bond between TyrZ and D1-His190 (~2.5 Å) Full size image W539 forms an H-bond with D1-Ser169 (O W539 –O D1-Ser169 = 2.73 Å), which has been proposed to provide access to water molecules for the substrate-binding site [42] . Incorporation of W539 into the O4 site was also observed in QM/MM calculations using the original PSII crystal structure and depleting the O4 atom (Fig. 6a ); the obtained geometry was consistent with the O4-incorporated geometry obtained through the S 2 , S 3 , and S 4 states (Fig. 4 ), which indicates the robustness of the present reaction scheme. Fig. 6 QM/MM geometries in the O4-depleted and O5-depleted PSII proteins. a Formation of the Mn3–O W539 and Mn4–O W539 bonds in response to incorporation of H 2 O at W539 into the O4 site of the O4-depleted Mn 4 CaO 4 cluster. b Shorting the Mn3–O W539 and Mn4–O W539 bonds in response to incorporation of H 2 O into the vacant W539 site. c QM/MM geometries in the O5-depleted PSII. (Mn1, Mn2, Mn3, Mn4) = (III, IV, III, III) Full size image As H 2 O at W539 was incorporated into the Mn 4 CaO 4 cluster, the W539 site became vacant. When the W539 site was refilled by a water molecule, both Mn3–O W539 and Mn4–O W539 were further shortened to ~2.2 Å (Fig. 6b ). It seems likely that incorporation of a water molecule via D1-Asp61 into the W539 site [16] led to fixation of O4 as a component of the Mn 4 CaO 5 cluster. Alteration of the H-bond pattern along the O4-water chain QM/MM calculations indicated that O4 may exist as OH – in S 0 , and release of the proton occurs in the S 0 -to-S 1 transition along the O4-water chain (Fig. 1 ), with transforming of the pre-PT to a post-PT H-bond pattern [4] . This implies that the pre-PT pattern must be recovered from the post-PT pattern before the next turnover. As W539 approached Mn3 during O 2 evolution, the H-bond pattern along the O4-water chain (e.g., W538) transformed from the post-PT pattern to the pre-PT pattern, since W539 (i.e., new O4) needs to reorient to form a μ-oxo bridge (Mn3–O W539 –Mn4) (Fig. 7 ). Given that release of the first proton from H 2 O at O4 occurs via D1-Asp61 in the pre-S 0 -to-S 0 transition (i.e., the O4-water chain is not used), the O4-water chain remains in the pre-PT pattern, ready for release of the proton in the S 0 -to-S 1 transition. Fig. 7 The energy profiles when W539 approaches Mn3(III). As W539 approaches Mn3(III) (i.e., the Mn3…O W539 distance was decreased), concertedly (1) W n -W1 approaches Mn4 (ligating to Mn4), (2) the H-bond pattern of the O4-water chain transforms from the post-PT to pre-PT pattern, and (3) O 2 releases from the Mn3 moiety. The total spin density 2 S is shown for O W1 =O4 Full size image The rate-limiting step in O=O formation has been reported to exhibit a k D / k H of 1.4 [6] , which is consistent with the k D / k H value for transformation between pre- and post-PT patterns [11] . This may correspond to H-bond transformation along the O4-water chain (Fig. 7 ), since the corresponding water chain or H-bond network is absent at the O5/O6 moiety [9] , [17] , [18] . Characteristic O sites in the two-flash structure The two-flash illuminated PSII structure shows the extremely short averaged O4…O W539 distance of 2.32 Å (2.47 and 2.17 Å) [17] . The present QM/MM calculations reproduced the short O4–O W539 distance (2.43 Å) when H 2 O at W539 was incorporated into the O4 site and the vacant W539 site was refilled by H 2 O (pre-S 0 state, Fig. 6b ). The absence of W538 (i.e., disordered W538) in the two-flash illuminated PSII structure [17] can be explained by the present reaction scheme, as O4 is consumed and thus incorporation of W539 and displacement of W538 occur (Fig. 6 ). The vacant W539-binding site (Fig. 6a ) can be refilled by H 2 O, as MD simulations indicated that bulk water could enter the W539 and W538 sites via D1-Asp61 [16] . Even in the Mn-depleted PSII crystal structure, both W539 and W538 exist and are well-ordered ( B -factor values are 33.9 and 43.4, respectively) [53] , highlighting the originally large binding affinity due to D1-Asp61. This, in turn, suggests that the absence of well-ordered W538 in the two-flash illuminated PSII structure [17] is exceptional (Table 2 ), and can be understood only when reorganization of W539 and W538 occurs. Table 2 B -factor values in the two-flash illuminated PSII structure (5WS6) and the 1.9-Å PSII structure (3ARC) (in Å 2 ) Full size table Based on the findings reported here, we are able to propose the following reaction scheme (Fig. 8 ). In S 2 , the H atom of H 2 O at W1 is significantly migrated toward D1-Asp61 in the open-cubane Mn(III,IV,IV,IV) (Fig. 2 ). The S 2 -to-S 3 transition involves oxidation of O W1 H – , resulting in formation of O W1 •– in Mn(III,IV,IV,IV), as suggested by Messinger et al. [32] . In S 3 , the binding of W1 at Mn4(IV) is pronounced due to formation of O W1 •– . The binding of W n -W1 at O W1 •– is also pronounced (Fig. 3 ). S 4 is initially Mn(IV,IV,IV,IV) with O W1 •– . Oxo-oxyl radical coupling between O4 and O W1 •– leads to formation of (O W1 –O4) 2– and reduction to Mn(IV,IV,III,IV) (Fig. 4 ); W n -W1 decreases the energy barrier for the (O W1 –O4) 2– formation, serving as a catalyst. As O W1 =O4 moves away from the Mn3/Mn4 moiety toward D1-Ile60 in the proposed O 2 -exiting pathway [48] , H 2 O at W539 is incorporated into the vacant O4 site, forming a μ-oxo bridge with Mn3–O W539 and Mn4–O W539 in a concerted exergonic process. W n -W1 is also incorporated into the Mn 4 CaO 5 cluster as the new W1 ligand. The two Mn3–O W539 and Mn4–O W539 bonds are further shortened when the vacant W539 site is refilled by a water molecule, which approaches via D1-Asp61 [16] , recovering the original Mn 4 CaO 5 structure. Incorporation of W539 into the O4 site also seems to lead to transformation of the H-bond pattern along the O4-water chain to the pre-PT pattern (Fig. 7 ), in readiness for proton transfer in the S 0 -to-S 1 transition [4] . Fig. 8 Mechanism of O 2 formation and recovery of Mn 4 CaO 5 . S 0 is the lowest oxidation state. In the S 0 -to-S 1 transition, a low-barrier H-bond between OH – at O4 and W539 (as indicated in the crystal structure [9] ) releases the proton via the O4-water chain [4] . In the O4-water chain, the pre-PT pattern transforms into the post PT pattern as a result of proton transfer. In the S 1 -to-S 2 transition, oxidation of Mn4(III) to Mn4(IV) occurs, resulting in a decrease in p K a of W1 and formation of a low-barrier H-bond between W1 and D1-Asp61. In the S 2 -to-S 3 transition, D1-Asp61 decreases the redox potential of W1 and facilitates proton-coupled oxidation of O W1 H – to O W1 •– . O W1 •– attracts W n -W1 . In S 4 , oxo-oxyl radical coupling occurs between O W1 •– and corner μ-oxo O4, leading to formation of (O W1 –O4) 2– , reduction of Mn, incorporation of W n -W1 as new W1, and approach of W539. In the S 4 -to-pre-S 0 transition, as O W1 =O4 moves away from the Mn 4 CaO 5 moiety, water incorporation occurs near two second sphere ligands, D1-Asp61 and CP43-Arg357: D1-Asp61 accepts an H-bond from W539 and incorporation of W539 into the vacant O4 site near CP43-Arg357 leads to reorientation of W539 and formation of a μ-oxo bridge with Mn3–O W539 and Mn4–O W539 . Reorientation of W539 (i.e., new O4) at the O4 site propagates along the O4-water chain, transforming the post-PT pattern to the pre-PT pattern. The vacant W539 site can be filled by a water molecule from the D1-Glu65/D2-Glu312 channel via D1-Asp61 [16] . Pre-S 0 , where H 2 O is present at O4, can be stabilized by release of a proton from the newly incorporated O4 site and proceeds to S 0 Full size image The proton releasing sites are identified as W1 in the S 2 -to-S 3 and the S 3 -to-S 0 transitions and O4 in the pre-S 0 -to-S 0 and S 0 -to-S 1 [4] transitions. Based on these observations, W1 and O4 are deprotonatable substrate water molecules on the current turnover, and W n -W1 and W539 serve as “holding sites [7] ” and become W1 and O4, respectively, on the next turnover. Then, the D1-Glu65/D2-Glu312 channel serves as a water intake channel for both substrate water molecules [16] . The location of O4/W539 at the dead end of the narrow region of the D1-Glu65/D2-Glu312 channel [16] may also make the exchange rate slow. If the fast-exchanging and slow-exchanging water molecules represent two substrate water molecules, they might be W1 and O4, respectively. 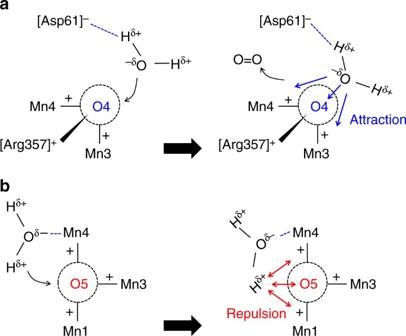Fig. 5 Difference in the orientations and interactions of the incorporating H2O molecule.aThe O4 site. Anionic D1-Asp61 attracts the Hδ+and orients the Oδ–of the incorporating H2O toward cationic Mn3(III), Mn4(III), and CP43-Arg357, resulting in attraction.bThe O5 site. The absence of an anionic H-bond acceptor and the nature of the incorporating H2O as a ligand of Mn4 force the Hδ+of the incorporating H2O to face cationic Mn1(III), Mn3(III), and Mn4(III), resulting in repulsion. The absence of D1-Asp61 near O5 would be energetically disadvantageous for incorporating H2O into the O5 site. O4 is located at the “corner” of the Mn3–O4 and O4–Mn4 bonds. Due to the presence of D1-Asp61, OW539δ–can always be oriented toward the vacant O4 site, which makes incorporation energetically favorable (Supplementary Figure4a). On the other hand, if W2 is incorporated into the center of the Mn1–(O5)–Mn4 bond, HW2δ+is oriented toward cationic Mn1(III) and Mn4(III), causing repulsion (Supplementary Figure4b). Indeed, QM/MM calculations show that neither W2 nor W3 was incorporated into the vacant O5 site of the O5-depleted Mn4CaO4cluster. Depletion of O5 did not even affect the H-bond network near O5, including the short low-barrier H-bond between TyrZ and D1-His190 (~2.5 Å) Then, the decrease in the exchange rate for the fast-exchanging water molecule in the S 2 -to-S 3 transition [12] might be explained by the pronounced binding of W1 at Mn4 (O W1 •– in S 3 ) (Supplementary Figure 5 ). However, as suggested by Noguchi and coworkers based on FTIR difference spectroscopy, it seems also possible that the exchanging water molecule is not necessarily a substrate water molecules on the current turnover (W1 and O4 in the present reaction scheme) but rather a substrate water molecule on the next turnover (W n -W1 as next W1 and W539 as next O4) [41] . In this case, the increase in the exchange rate of the slow-exchanging water molecule (i.e., W539) in the S 1 -to-S 2 transition [12] is due to the relaxed H-bond network of the O4-water chain (including O4 and W539) in the S 1 -to-S 2 transition (i.e., after proton transfer) with respect to the strongly coupled H-bond network in the S 0 -to-S 1 transition [4] . The decrease in the exchange rate for the fast-exchanging water molecule (i.e., W n -W1 ) in the S 2 -to-S 3 transition [12] can be explained by the pronounced binding of W n -W1 at O W1 •– . W n -W1 , a substrate on the next turnover, decreases the energy barrier for (O W1 –O4) 2– formation in S 4 , serving as a catalyst. W539, another substrate on the next turnover, is the direct proton acceptor for the current turnover substrate H 2 O at O4. The remarkable cooperativity of the next substrate water molecules to catalyze the current substrate water molecule (Fig. 4b ), as well as the self-recovery of the Mn 4 CaO 5 cluster from the O 2 -evolved Mn 4 CaO 4 cluster in a concerted exergonic process (Fig. 4a ), suggest that W1/ W n -W1 and O4/W539 are substrate water molecules. Coordinates and atomic partial charges The atomic coordinates of PSII were taken from the X-ray structure of PSII monomer unit “A” of the PSII complexes from Thermosynechococcus vulcanus at a resolution of 1.9 Å (PDB code, 3ARC) [9] . During optimization of hydrogen atom positions with CHARMM [54] , the positions of all heavy atoms were fixed and all titratable groups (e.g., acidic and basic groups) were ionized. In QM/MM calculations, additional counter ions were added to neutralize the entire system. Atomic partial charges of the amino acids and cofactors were obtained from the CHARMM22 [55] parameter set and our previous studies on PSII [4] , respectively. D1-His337 was considered to be protonated [56] . QM/MM calculations The unrestricted density functional theory (DFT) method was employed with the B3LYP functional and LACVP* basis sets, using the QSite [57] program. In the QM region, all the atomic coordinates were fully relaxed. In the MM region, the positions of H atoms were optimized using the OPLS2005 force field, while the positions of heavy atoms were fixed. The cluster was considered to be in the S 2 , S 3 , S 4 , and S 0 states with antiferromagnetically coupled Mn ions; the resulting Mn oxidation states (Mn1, Mn2, Mn3, Mn4) and the total spin S were as follows: (III, IV, IV, IV) and S = 7/2 (↑↓↑↑) in S 2 ; (III, IV, IV, IV) + O W1 •– and S = 8/2 (↑↓↑↑ + ↑) in S 3 ; (IV, IV, IV, IV) + O W1 •– and S = 7/2 (↑↓↑↑ + ↑), (IV, IV, III, IV) + (O W1 –O4) 2– and S = 7/2 (↑↓↑↑), and (III, IV, III, III) + O W1 =O4 and (↑↓↑↑ + ↓) in S 4 ; (III, IV, III, III) and S = 9/2 (↑↓↑↑) in pre-S 0 (Table 1 , Supplementary Figures 1 and 3 for other spin configurations). The Mn 4 CaO 5 geometry in S n was obtained as follows: first we prepared the QM/MM-optimized S n geometry with ferromagnetically coupled Mn ions, using the QM/MM-optimized S n –1 geometry. The resulting S n geometry was then optimized as antiferromagnetically coupled Mn ions. The initial-guess wave functions were obtained by using the ligand-field theory [58] implemented in the QSite program. See Supplementary Data 1 for the atomic coordinates. To analyze S 2 , S 3 (Fig. 2 ), and S 4 (Fig. 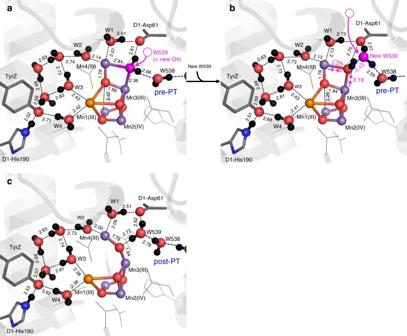Fig. 6 QM/MM geometries in the O4-depleted and O5-depleted PSII proteins.aFormation of the Mn3–OW539and Mn4–OW539bonds in response to incorporation of H2O at W539 into the O4 site of the O4-depleted Mn4CaO4cluster.bShorting the Mn3–OW539and Mn4–OW539bonds in response to incorporation of H2O into the vacant W539 site.cQM/MM geometries in the O5-depleted PSII. (Mn1, Mn2, Mn3, Mn4) = (III, IV, III, III) 4 ), the QM region (small QM) was defined as the Mn 4 CaO 5 cluster (including the ligand side-chains of D1-Asp170, D1-Glu189, D1-His332, D1-Glu333, D1-Asp342, and CP43-Glu354, and the backbone of D1-Ala344); the ligand water molecules of W1-W4; the O4-water chain (W539, W538, and W393); the W n -W1 -binding site (W n -W1 , W426, and W614); the Cl-1-binding site (Cl-1, W442, W446, and side-chains of D1-Asn181 and D2-Lys317); and the second sphere ligands (side-chains of D1-Asp61 and CP43-Arg357). Other groups were approximated by the MM force field. To mainly analyze the O4-depleted and O5-depleted PSII structures in S 0 (Fig. 6 ), the QM region (large QM) was defined as the Mn 4 CaO 5 cluster (including the ligand side-chains of D1-Asp170, D1-Glu189, D1-His332, D1-Glu333, D1-Asp342, and CP43-Glu354, and the backbone of D1-Ala344); the ligand water molecules of W1-W4; the O4-water chain (W539); the Cl-1-binding site (Cl-1, W442, W446, and side-chains of D1-Asn181 and D2-Lys317); the second sphere ligands (side-chains of D1-Asp61 and CP43-Arg357); the H-bond network of TyrZ (side-chains of D1-Tyr161, D1-His190, and D1-Asn298), and the diamond-shaped cluster of water molecules [59] (W5, W6, and W7). To obtain the potential-energy profiles of H-bonds (Fig. 2b and Supplementary Fig. 1 ), the QM/MM optimized geometry was used as the initial geometry. The H atom under investigation was moved from the H-bond donor atom (O donor ) toward the acceptor atom (O acceptor ) by 0.05 Å, after which the geometry was optimized by constraining the O donor –H and H–O acceptor distances and the energy was calculated. This procedure was repeated until the H atom reached the O acceptor atom. To obtain the potential-energy profiles of (O W1 –O4) 2– formation (Fig. 4b and Supplementary Fig. 3 ) and O 2 release (Fig. 7 and Supplementary Fig. 4 ), the QM/MM optimized geometry was used as the initial geometry; e.g., the O W1 …O4 distance was then decreased by 0.05 Å, after which the geometry was optimized by constraining the O W1 …O4 distance and the energy was calculated. 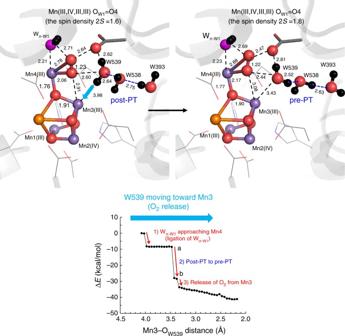Fig. 7 The energy profiles when W539 approaches Mn3(III). As W539 approaches Mn3(III) (i.e., the Mn3…OW539distance was decreased), concertedly (1) Wn-W1approaches Mn4 (ligating to Mn4), (2) the H-bond pattern of the O4-water chain transforms from the post-PT to pre-PT pattern, and (3) O2releases from the Mn3 moiety. The total spin density 2Sis shown for OW1=O4 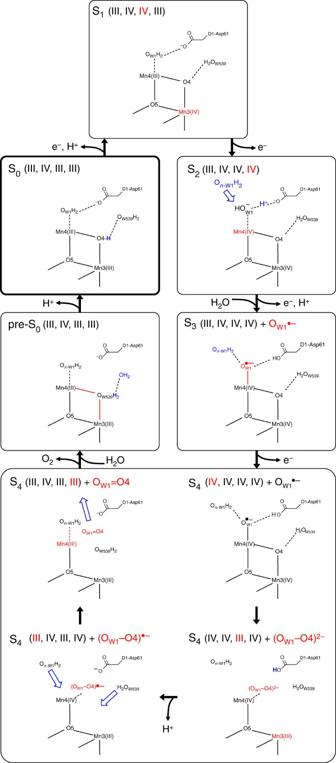Fig. 8 Mechanism of O2formation and recovery of Mn4CaO5. S0is the lowest oxidation state. In the S0-to-S1transition, a low-barrier H-bond between OH–at O4 and W539 (as indicated in the crystal structure9) releases the proton via the O4-water chain4. In the O4-water chain, the pre-PT pattern transforms into the post PT pattern as a result of proton transfer. In the S1-to-S2transition, oxidation of Mn4(III) to Mn4(IV) occurs, resulting in a decrease in pKaof W1 and formation of a low-barrier H-bond between W1 and D1-Asp61. In the S2-to-S3transition, D1-Asp61 decreases the redox potential of W1 and facilitates proton-coupled oxidation of OW1H–to OW1•–. OW1•–attracts Wn-W1. In S4, oxo-oxyl radical coupling occurs between OW1•–and corner μ-oxo O4, leading to formation of (OW1–O4)2–, reduction of Mn, incorporation of Wn-W1as new W1, and approach of W539. In the S4-to-pre-S0transition, as OW1=O4 moves away from the Mn4CaO5moiety, water incorporation occurs near two second sphere ligands, D1-Asp61 and CP43-Arg357: D1-Asp61 accepts an H-bond from W539 and incorporation of W539 into the vacant O4 site near CP43-Arg357 leads to reorientation of W539 and formation of a μ-oxo bridge with Mn3–OW539and Mn4–OW539. Reorientation of W539 (i.e., new O4) at the O4 site propagates along the O4-water chain, transforming the post-PT pattern to the pre-PT pattern. The vacant W539 site can be filled by a water molecule from the D1-Glu65/D2-Glu312 channel via D1-Asp6116. Pre-S0, where H2O is present at O4, can be stabilized by release of a proton from the newly incorporated O4 site and proceeds to S0 This procedure was repeated until formation of (O W1 –O4) 2– . MD simulations The PSII structure was embedded in a lipid bilayer, which is composed of 546 1-palmitoyl-2-oleyl-sn-glycero-3-phosphocholine (POPC), and soaked in 78889 flexible water molecules (SPC-Fw) [60] , using the CHARMM-GUI program [61] . After geometry optimization with position restraints on heavy atoms, the system was heated from 0.001 K to 300 K during 5.0 ps. The position restraints on heavy atoms were gradually released over 16.5 ns. An equilibrating MD run was conducted for 45 ns using the MD engine AMBER 14 [62] with the SHAKE algorithm for hydrogen constraint [63] . The production run was conducted with an MD time step of 0.5 fs without hydrogen constraint, using AMBER 14. To control temperature and pressure, the Berendsen thermostat and barostat were employed [65] . See ref. [16] for force field parameters. Data availability All the data supporting the findings of this study are available within the article and its Supplementary Information files or from the corresponding author upon reasonable request.